Translocation path of a substrate protein through its Omp85 transporter TpsB proteins are Omp85 superfamily members that mediate protein translocation across the outer membrane of Gram-negative bacteria. Omp85 transporters are composed of N-terminal POTRA domains and a C-terminal transmembrane β-barrel. In this work, we track the in vivo secretion path of the Bordetella pertussis filamentous haemagglutinin (FHA), the substrate of the model TpsB transporter FhaC, using site-specific crosslinking. The conserved secretion domain of FHA interacts with the POTRA domains, specific extracellular loops and strands of FhaC and the inner β-barrel surface. The interaction map indicates a funnel-like pathway, with conformationally flexible FHA entering the channel in a non-exclusive manner and exiting along a four-stranded β-sheet at the surface of the FhaC barrel. This sheet of FhaC guides the secretion domain of FHA along discrete steps of translocation and folding. This work demonstrates that the Omp85 barrel serves as a channel for translocation of substrate proteins. The widespread ‘two-partner secretion’ (TPS) pathway mediates the translocation of large proteins, involved in adherence, cytolysis, iron acquisition or growth inhibition, across the outer membrane of both pathogenic and non-pathogenic Gram-negative bacteria [1] . TPS systems are composed of two proteins, collectively called ‘TpsA’ for the secretory proteins and ‘TpsB’ for their transporters [2] . The secreted TspA proteins share a conserved, 250-residue-long N-terminal ‘TPS’ domain essential for secretion and a β-helix fold [3] , [4] , [5] , [6] , [7] . TpsB transporters are integral outer membrane proteins of the Omp85 superfamily, which is found in all branches of the phylogenetic tree [8] . Omp85 transporters mediate the translocation of their protein substrate(s) across, or their assembly into, specific cellular membranes. They share a common architecture that consists of a transmembrane β-barrel domain preceded by one or several POTRA domain(s) located in the inter-membrane space [9] , [10] , [11] , [12] . The POTRA domains appear to mediate protein–protein interactions [13] , [14] , [15] , [16] . However, the molecular mechanisms of protein transport or integration and in particular the role of the β-barrel remain poorly understood [11] , [12] , [17] , [18] , [19] , [20] , [21] . The filamentous haemagglutinin (FHA)/FhaC system of the whooping cough agent, Bordetella pertussis , is a model for the TPS pathway. The TpsA protein FHA, a major adhesin of B. pertussis [22] , is translocated to the bacterial surface by its TpsB partner, FhaC. The crystal structures of Fha30, a 30-kDa secretion-competent N-terminal FHA truncated fragment, and of FhaC have been determined [4] , [9] . Fha30 comprises the entire TPS domain of FHA, which forms a right-handed, parallel β-helix flanked by conserved anti-parallel β-structure elements, and a few additional β-helix coils after the TPS domain [4] ( Fig. 1a ). FhaC is composed of two periplasmic POTRA domains in tandem followed by a 16-stranded transmembrane β-barrel [9] ( Fig. 1b ). The pore of the barrel is obstructed by the N-terminal α-helix H1 and the extracellular loop L6 of FhaC. H1 is joined to the barrel-distal POTRA1 domain by a 25-residue-long periplasmic linker. We have recently shown that H1 is mobile within the pore and can move to the periplasm [23] . The extracellular loop L6, which folds back into the pore, harbours a conserved sequence motif characteristic of the Omp85 superfamily and is essential for function [9] , [24] , [25] , [26] . According to the current secretion model, FhaB, the FHA precursor, is exported across the cytoplasmic membrane by the Sec machinery and chaperoned by DegP in the periplasm [27] , [28] , [29] . The POTRA domains of FhaC recognize the TPS domain of FHA in an extended conformation, leading to the translocation of the secretory polypeptide across the outer membrane [14] , [30] , [31] . Whether FHA transport occurs through the pore of the FhaC β-barrel has not been shown. Upon secretion, FHA folds progressively into a long β-helix at the cell surface before undergoing a proteolytic maturation that partially releases it into the milieu [32] . 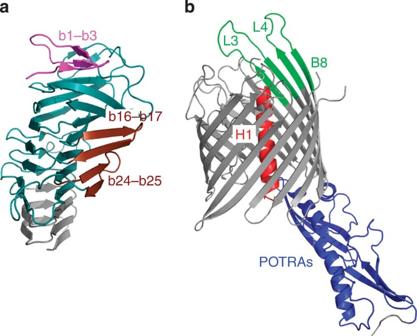Figure 1: Structures of Fha30 and FhaC. Cartoon representation of Fha30 (protein data bank: 1rwr,a) and FhaC (protein data bank: 2qdz,b). In Fha30, the TPS domain is coloured while the additional β-strands are in grey. The strands that form extra-β-helix elements in the TPS domain have been indicated with small ‘b’ letters to distinguish them from the FhaC strands (capital ‘B’ letters) discussed in the text. Note that in the X-ray structure of FhaC, the linker and L5 are not resolved. The figures were created with Pymol. Figure 1: Structures of Fha30 and FhaC. Cartoon representation of Fha30 (protein data bank: 1rwr, a ) and FhaC (protein data bank: 2qdz, b ). In Fha30, the TPS domain is coloured while the additional β-strands are in grey. The strands that form extra-β-helix elements in the TPS domain have been indicated with small ‘b’ letters to distinguish them from the FhaC strands (capital ‘B’ letters) discussed in the text. Note that in the X-ray structure of FhaC, the linker and L5 are not resolved. The figures were created with Pymol. Full size image In this work, we track the translocation path of FHA across the outer membrane by performing in vivo , cysteine-directed crosslinking. We show that the β-barrel of FhaC serves as the protein-conducting channel. An extracellular β-sheet of FhaC is crucial for function, and translocation of the TPS domain proceeds by discrete steps. Mapping of FhaC regions that interact with FHA To map the regions of FhaC that are in contact with FHA during secretion, we looked for a model substrate that crosses the outer membrane in an FhaC-dependent manner and folds independently of the rest of FHA [4] , [30] , which is produced at good levels in Escherichia coli , and that interacts long enough with FhaC for detectable inter-protein crosslinking to occur. Although Fha30, a secretion-competent, N-terminal truncated fragment of FHA, met the first conditions [4] , initial experiments with nonspecific crosslinkers indicated that it was secreted much too fast. Thus, to freeze the interactions between the two partners, we used the Fha30-BugE chimaera [23] . When co-produced with FhaC in E. coli , this chimaera stalls across the outer membrane, with its Fha30 moiety exposed to the cell surface and the globular BugE moiety in the periplasm. We have shown that such chimaeras mimic translocation intermediates and can thus be used as tools to probe the on-going secretion process [23] . Single Cys residues were introduced at >50 positions in FhaC by site-directed mutagenesis ( Fig. 2a ). The substitutions did not affect the production of FhaC, its location in the outer membrane or its ability to secrete Fha30 ( Supplementary Fig. 1 ). We co-produced Fha30-BugE with each FhaC Cys variant in E. coli . In this system, the expression of FhaC is under the control of a weak constitutive promoter, while that of the chimaera is induced with isopropyl-β- D -thiogalactoside (IPTG) for a short period of time at the exponential growth phase of the culture, so that the chimaera is presented to preformed FhaC in the outer membrane. The bacteria were treated with the heterofunctional sulfhydryl-to-amine crosslinkers SPDP (succinimidyl 3-(2-pyridyldithio) propionate), LC-SPDP (long chain SPDP)or SMCC (succinimidyl 4-(N-maleimidomethyl)cyclohexane-1-carboxylate), and following disruption of the bacterial membranes, FhaC- or FhaC-containing complexes were isolated by taking advantage of the property of FhaC to bind to Ni ++ beads irrespective of a 6-His tag. The material eluted from the beads was analysed by immunoblotting using anti-Fha30 and anti-FhaC antibodies ( Fig. 2b and Supplementary Fig. 2 ). Complexes between the two proteins were detected for FhaC derivatives harbouring Cys residues in the POTRA domains, a periplasmic loop, the barrel interior (B9–B11), the extracellular portions of β-strands B5, B7 and B8, and the extracellular loops L3, L4 and L5, but not in H1, the linker, other extracellular loops or in a lipid-facing position of the β-barrel (Cys468). Low amounts of crosslinked species were also found for some FhaC variants with Cys residues in the conserved L6 loop. 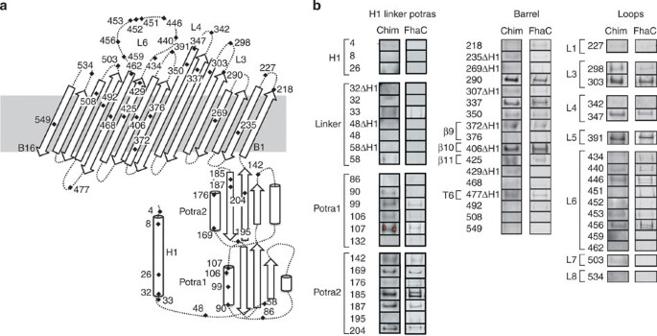Figure 2: Crosslinking analyses with FhaC Cys variants. (a) Schematic representation of the FhaC topology, with the positions of the Cys residues introduced for crosslinking experiments indicated as black diamonds. The topology is based on a slightly revised version of the FhaC structure (protein data bank: 4qky). (b) Immunoblot analyses of the SMCC-crosslinked complexes or the SPDP-crosslinked complexes for the FhaCΔH1Cys429and FhaCΔH1Cys372variants following precipitation of FhaC. The membranes were probed successively with anti-Fha30 antibodies followed by chemiluminescence detection, and with anti-FhaC antibodies followed by alkaline phosphatase detection. The crosslinked complex migrates slightly under the 150-kDa band of the molecular mass markers that is indicated by a small horizontal dash at the left of the first subpanel. Note the presence of two FhaC-containing bands in some cases, the upper one corresponding to the complex and the other to an FhaC dimer that most likely formed upon cell lysis. Some FhaC variants with Cys in the barrel were devoid of H1 to facilitate crosslinker access (denoted as ΔH1), since H1 is not essential for activity37and moves to the periplasm for FHA translocation23. We checked for one such variant, FhaCC406, that similar results were obtained with or without H1. In the β-barrel, we mainly selected residues oriented towards the pore based on the crystal structure of FhaC. Lipid-oriented residue 468 was used as a control. Figure 2: Crosslinking analyses with FhaC Cys variants. ( a ) Schematic representation of the FhaC topology, with the positions of the Cys residues introduced for crosslinking experiments indicated as black diamonds. The topology is based on a slightly revised version of the FhaC structure (protein data bank: 4qky). ( b ) Immunoblot analyses of the SMCC-crosslinked complexes or the SPDP-crosslinked complexes for the FhaCΔH1 Cys429 and FhaCΔH1 Cys372 variants following precipitation of FhaC. The membranes were probed successively with anti-Fha30 antibodies followed by chemiluminescence detection, and with anti-FhaC antibodies followed by alkaline phosphatase detection. The crosslinked complex migrates slightly under the 150-kDa band of the molecular mass markers that is indicated by a small horizontal dash at the left of the first subpanel. Note the presence of two FhaC-containing bands in some cases, the upper one corresponding to the complex and the other to an FhaC dimer that most likely formed upon cell lysis. Some FhaC variants with Cys in the barrel were devoid of H1 to facilitate crosslinker access (denoted as ΔH1), since H1 is not essential for activity [37] and moves to the periplasm for FHA translocation [23] . We checked for one such variant, FhaC C406 , that similar results were obtained with or without H1. In the β-barrel, we mainly selected residues oriented towards the pore based on the crystal structure of FhaC. Lipid-oriented residue 468 was used as a control. Full size image Thus, three regions of FhaC principally interact with the stalled Fha30-BugE chimaera: the surface of the POTRA domains oriented towards the β-barrel, the inner wall of the barrel, and specific extracellular loops and strands. Detection of crosslinks between the chimaera and inward-facing residues of the FhaC β-barrel strands B9–B11 located halfway into the pore ( Fig. 2 ) provides the first direct evidence that the TpsA protein crosses the outer membrane through the proteinaceous channel formed by its TpsB partner. In addition, most FhaC–chimaera crosslinks involving extracellular portions of FhaC are localized in an extracellular β-sheet formed by the longest β-barrel strands (B5–B8) and in nearby surface loops L3, L4 and L5. As for the interactions of the POTRA domains with the chimaera, they involve the same regions of the POTRA domains as those identified to interact with Fha30 in vitro [14] . The topology of the chimaera suggests that BugE, rather than Fha30, is in contact with the POTRA domains in these stalled complexes. To confirm the pathway observed with Fha30-BugE and to ascertain that it was not affected by the presence of the BugE cargo, we performed a limited number of crosslinking experiments with another model substrate harbouring a different cargo, Fha30-calmo. Of note, we have shown that this chimaera could be released into the milieu from the stalled complex after unfolding its calmodulin cargo [23] . The Fha30-calmo chimaera was found to crosslink with FhaC in a similar manner as the Fha30-BugE model substrate, although the amounts of complex were weaker ( Supplementary Fig. 3 ). Regions of FHA that interact with FhaC To identify regions of the TPS domain that are close to FhaC in the course of translocation, we introduced Cys residues at various positions of the Fha30 moiety of the Fha30-BugE chimaera ( Fig. 3a and Supplementary Table 1 for the list of positions tested). In addition to a few β-helix positions, we particularly targeted segments that form extra-β-helix elements conserved in the TpsA family [4] , [5] , [6] . Most substitutions do not affect the secretion of Fha30 alone, enabling us to use the corresponding chimaeras for crosslinking, while those that abolish secretion or cause intracellular proteolytic degradation of the chimaera were discarded ( Supplementary Table 1 ). In vivo crosslinking experiments showed that Cys residues in two major discrete regions of the TPS domain mediate the formation of complexes between the chimaera and FhaC: the N-terminal region up to b8, and the region encompassing residues 176–200 in the second part of the TPS domain, that is, in the less conserved ‘LC2’ region [4] ( Fig. 3b and Supplementary Fig. 4 ). 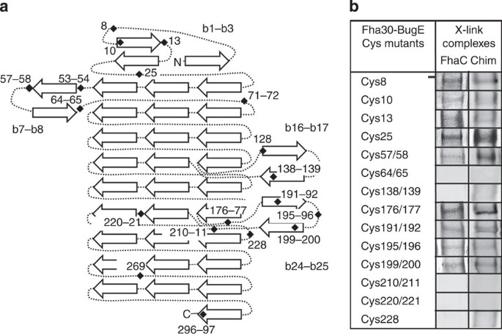Figure 3: Crosslinking analyses with Fha30-BugE Cys variants. (a) Schematic representation of the Fha30 topology, with the positions of the Cys residues introduced for crosslinking experiments indicated as black diamonds. (b) Immunoblot analyses of the SMCC-crosslinked complexes or the LC-SPDP-crosslinked complexes for the chimaera Cys13, Cys191/192 and Cys199/200 variants following precipitation of FhaC. The membranes were probed successively with anti-Fha30 antibodies and with anti-FhaC antibodies as above. The crosslinked complex migrates slightly under the 150-kDa band of the markers that is indicated by a short horizontal dash at the left of the first subpanel. Figure 3: Crosslinking analyses with Fha30-BugE Cys variants. ( a ) Schematic representation of the Fha30 topology, with the positions of the Cys residues introduced for crosslinking experiments indicated as black diamonds. ( b ) Immunoblot analyses of the SMCC-crosslinked complexes or the LC-SPDP-crosslinked complexes for the chimaera Cys13, Cys191/192 and Cys199/200 variants following precipitation of FhaC. The membranes were probed successively with anti-Fha30 antibodies and with anti-FhaC antibodies as above. The crosslinked complex migrates slightly under the 150-kDa band of the markers that is indicated by a short horizontal dash at the left of the first subpanel. Full size image Tracking the FHA path in FhaC Next, we combined single Cys variants of FhaC with those of Fha30-BugE, and looked for spontaneous formation of inter-protein disulfide (S–S) bonds in the course of translocation in order to obtain a site-specific interaction map. N-ethyl maleimide was added before cell lysis to avoid extraneous bonds. A number of specific FhaC–chimaera complexes were detected ( Fig. 4 , Supplementary Table 2 and Supplementary Fig. 5 ). Positions up to b16–b17 in Fha30 formed S–S bonds with the POTRA domains of FhaC, as well as with the linker. In addition, several regions of FHA including the b7, b8, b24 and b25 strands formed S–S bonds with the barrel interior. Finally, the N-terminal cap (b1–b3) and a central region of the TPS domain (residues 191–221) both formed crosslinks with the extracellular sheet of FhaC ( Fig. 4 , Supplementary Table 2 ). Altogether, there is a good agreement between the chemical crosslinks and the spontaneous S–S bonds. 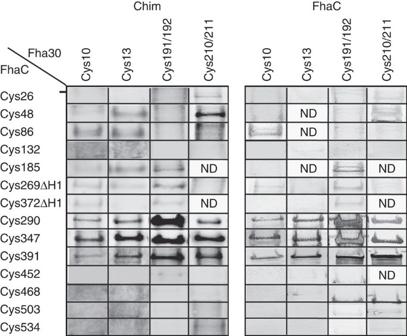Figure 4: Spontaneous formation of S–S bonds between FhaC and Fha30-BugE. The membranes were successively probed with anti-Fha30 antibodies followed by chemiluminescence detection (left panel), and with anti-FhaC antibodies followed by alkaline phosphatase detection (right panel). The crosslinked complex migrates slightly under the 150-kDa band of the markers that is indicated by a short horizontal dash at the left of the first subpanel. ND, not determined. Figure 4: Spontaneous formation of S–S bonds between FhaC and Fha30-BugE. The membranes were successively probed with anti-Fha30 antibodies followed by chemiluminescence detection (left panel), and with anti-FhaC antibodies followed by alkaline phosphatase detection (right panel). The crosslinked complex migrates slightly under the 150-kDa band of the markers that is indicated by a short horizontal dash at the left of the first subpanel. ND, not determined. Full size image In many cases, a given Cys in Fha30 was involved in S–S bonds with several Cys residues located in non-contiguous regions of FhaC ( Supplementary Table 2 ), indicating sequential or alternative interactions of the secretory polypeptide with its transporter. In particular, each of the three N-proximal Cys of Fha30 crosslinked with the POTRA domains, the inner barrel surface, the extracellular β-strands B5–B8 and the L5 loop. These interactions thus track possible paths of the Fha30 N terminus through FhaC. The observation that some Fha30 Cys residues (for example, Cys8 or Cys190/191) formed S–S bonds with opposite sites in the first half of the barrel (Cys269 in B4 and Cys372 in B9) indicates that the chimaera does not enter the FhaC channel along a strictly defined path. Instead, it appears to interact by >1 manner with the entrance of the FhaC channel. In contrast, interactions at the exit of the channel involved principally one side of the barrel, with intense S–S-bonded complexes involving B5–B8 (Cys290, Cys337 and Cys347) and L5 (Cys391) of FhaC, and N-terminal (Cys8 and Cys25) and central (residues 190–221) regions of Fha30. Interestingly, these two regions harbour non-β-helix, anti-parallel structural elements in the native TPS domain, including the b1–b3 cap of the β-helix and the b24–b25 β-hairpin ( Fig. 1a ). Identification of putative translocation intermediates Two regions that are not spatially close to each other in Fha30—that is, the N-terminal region and a central region of the TPS domain—both interact with the extracellular B5–B8 β sheet of FhaC. Therefore, we hypothesized that these interactions reflect sequential intermediates of translocation captured by crosslinking because they correspond to translocation pauses. This was tested by treating bacteria that co-produce Fha30-BugE and FhaC with proteinase K without any crosslinking. This was done on intact or outer membrane-permeabilized bacteria. BugE in the chimaera was tagged with a C-terminal myc epitope for detection ( Fig. 5 ). Cell samples were precipitated with trichloroacetic acid (TCA), and the chimaera fragments were detected by immunoblotting with anti-Fha30 or anti-myc antibodies. 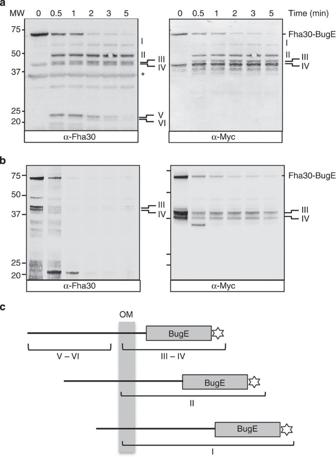Figure 5: Identification of translocation intermediates by proteolysis. Intact (a) or permeabilized (b) cells co-expressing Fha30-BugE with a C-terminal myc tag and FhaC were treated with proteinase K for the indicated times. Neither protein harboured a Cys residue and no chemical cross-linker was added. After TCA precipitation, total cellular proteins were analysed by immunoblotting using anti-Fha30 (left panels) or anti-myc (right panels) antibodies. The asterisk indicates a nonspecific band. A schematic representation of the chimaera and its proteolytic fragments is shown inc. OM and the grey rectangle denote the outer membrane. Figure 5: Identification of translocation intermediates by proteolysis. Intact ( a ) or permeabilized ( b ) cells co-expressing Fha30-BugE with a C-terminal myc tag and FhaC were treated with proteinase K for the indicated times. Neither protein harboured a Cys residue and no chemical cross-linker was added. After TCA precipitation, total cellular proteins were analysed by immunoblotting using anti-Fha30 (left panels) or anti-myc (right panels) antibodies. The asterisk indicates a nonspecific band. A schematic representation of the chimaera and its proteolytic fragments is shown in c . OM and the grey rectangle denote the outer membrane. Full size image Treatment of intact cells yielded species of ~60, 50 and 45 kDa that reacted with both antibodies (denoted I–IV) and shorter species ~22–23 kDa (V and VI) detected only with anti-Fha30 antibodies ( Fig. 5a,c ). In permeabilized cells, bands I and II disappeared, and species slightly smaller than III and IV were only detected with the anti-myc antibodies ( Fig. 5b,c ). This indicated that BugE is resistant to proteolysis, while Fha30 portions in species I and II are protected from degradation by the outer membrane in intact cells but mostly degraded after permeabilization. Species V and VI most likely encompass surface-exposed Fha30 fragments fairly resistant to protease treatment. The low-abundance species detected by immunoblotting could not be identified by mass fingerprinting analyses from total cell lysates. To confirm the identity of species V and VI, we treated purified Fha30 with proteinase K and analysed the polypeptides by mass fingerprinting ( Supplementary Fig. 6 ). The major proteolytic product of native Fha30 that most likely corresponds to species V or VI encompasses the N-terminal two-thirds of Fha30. Altogether, thus, the presence of species I–IV confirms the occurrence of intermediates of translocation, which is consistent with the idea that secretion proceeds by steps. Role of extracellular β-sheet of FhaC Finally, to probe the importance of the extracellular B5–B8 β-sheet for FhaC secretion activity, we deleted the L3 and L4 loops and shortened the extracellular portions of the B5–B8 β-strands. The FhaC variants were detected in normal amounts in the cells, but secretion was affected or abolished by these deletions, unlike for the L1 or L2 deletion variants used as controls ( Fig. 6a ). Consistent with this secretion defect, low amounts of cell-associated Fha30-BugE were found, indicating significant intracellular degradation of the chimaera. Integrity of the extracellular B5–B8 sheet and of the L3 and L4 loops is thus important for FhaC function. 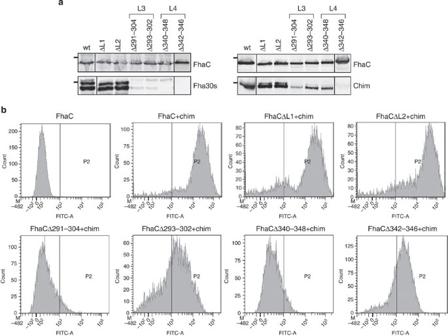Figure 6: Importance of the extracellular β sheet B5–B8 for FhaC activity. (a) Effects of deletions in the L3 and L4 loops on Fha30 secretion (denoted as Fha30s) and on the presence of cell-associated FhaC and Fha30-BugE (denoted as chim). Culture supernatants of cells co-producing FhaC and Fha30 (left panel), or lysates of cells co-producing FhaC and Fha30-BugE (right panel) were analysed by immunoblotting with anti-FhaC and anti-Fha30 antibodies. FhaC, Fha30 and Fha30-BugE chimaera migrate below the 75-kDa band of the markers, slightly below the 37-kDa band and slightly below the 75-kDa band, respectively, as indicated by short horizontal dashes at the left of the respective panels. (b) Flow cytometry analyses ofE. colico-expressing Fha30-BugE with an N-terminal myc tag and selected FhaC variants. Exposure of the Fha30 moiety of the chimaera at the cell surface was revealed using an anti-myc fluorescein isothiocyanate (FITC)-conjugated antibody. Wt, wild type. Figure 6: Importance of the extracellular β sheet B5–B8 for FhaC activity. ( a ) Effects of deletions in the L3 and L4 loops on Fha30 secretion (denoted as Fha30s) and on the presence of cell-associated FhaC and Fha30-BugE (denoted as chim). Culture supernatants of cells co-producing FhaC and Fha30 (left panel), or lysates of cells co-producing FhaC and Fha30-BugE (right panel) were analysed by immunoblotting with anti-FhaC and anti-Fha30 antibodies. FhaC, Fha30 and Fha30-BugE chimaera migrate below the 75-kDa band of the markers, slightly below the 37-kDa band and slightly below the 75-kDa band, respectively, as indicated by short horizontal dashes at the left of the respective panels. ( b ) Flow cytometry analyses of E. coli co-expressing Fha30-BugE with an N-terminal myc tag and selected FhaC variants. Exposure of the Fha30 moiety of the chimaera at the cell surface was revealed using an anti-myc fluorescein isothiocyanate (FITC)-conjugated antibody. Wt, wild type. Full size image Flow cytometry analyses were performed on cells co-producing Fha30-BugE that harbours an N-terminal myc tag and the FhaC variants ( Fig. 6b ). The bacteria were treated with an anti-myc fluorescein isothiocyanate conjugate for detection of the chimaera at the surface. Cells that produced the FhaC variants with the longer deletions showed no labelling at all, indicating that they could not translocate the chimaera, consistent with its intracellular degradation. The other bacteria were labelled by the antibody at lower levels than controls ( Fig. 6b ). Alterations of the B5–B8 β sheet thus prevent the chimaera from engaging properly into the channel and/or from stably reaching the cell surface, which strongly compromises secretion. Thus, the extracellular β-sheet of FhaC is a critical determinant for activity. In this work, we use the model FHA/FhaC TPS system to define the pathway of the secreted TpsA protein across its outer membrane transporter TpsB. By freezing the interactions between the partners, we characterize them during translocation and provide here the first evidence of an Omp85 substrate using the β-barrel of its transporter as a channel. Spontaneous S–S bond formation between the two proteins in the course of secretion also provides a dynamic view with snapshots of the transport process. We uncover the critical role of an extracellular β-sheet for FhaC secretion activity. Interestingly, corresponding surface regions of the E. coli Omp85 transporter BamA were also found to be essential for function [33] , [34] . In the crystal structure, the FhaC channel is mostly obstructed by the N-terminal α-helix H1 (ref. 9 ). Our findings that FHA threads its way through the FhaC pore is consistent with our findings that H1 plugs the resting barrel and moves to the periplasm for FHA translocation [23] . L6 is also located in the β-barrel pore of Omp85 transporters [9] , [11] , [12] . Unlike H1, however, we do not know whether it fully moves out of the FhaC pore in the course of secretion. The drastic effects of deletions, amino-acid substitutions and the observation of conformational changes have suggested that L6 participates in the transport mechanism of Omp85 proteins [11] , [21] , [26] , [35] , [36] . Our findings that L6 of FhaC weakly interacts with the substrate in the course of translocation argue against its playing a direct role to pull the secretory polypeptide towards the surface. How it contributes to activity remains a major unanswered question for Omp85 transporters. The four-stranded B5–B8 surface β-sheet of FhaC strongly interacts with FHA in the course of translocation. Its structural integrity is critical for FhaC function, as shown by the drastic effects of deletions. In support of this, we showed earlier that insertions in B5, B6 and L4 inactivated FhaC [35] , [37] . Notably, B5–B8 are generally long, and B9 is short in TpsB proteins ( Supplementary Fig. 7 ). In addition, the available Omp85 structures show that the B5–B8 β sheet is a conserved structural feature of the β-barrel [9] , [11] , [12] , [34] . These observations support a specific role for this sheet in the transport mechanism. In FhaC, B5–B8 appears to serve as a guide to which specific portions of the TPS domain bind in the course of translocation. This binding might involve β-augmentation of the edge strand of the FhaC β-sheet. In BamA, the extracellular loops L3 and L4 that join B5 to B6 and B7 to B8 form a dome over the barrel together with two other surface loops, thus limiting the opening of the channel to the milieu [11] , [34] . In the E. coli BamA, L3 also delineates with other loops a hydrophilic surface cavity proposed to facilitate the transport of soluble loops or domains of the substrate proteins [34] . Thus, the distinct conformations of these extracellular regions in FhaC and BamA are in good agreement with the respective functions of the two types of transporters. The preferential crosslinks of two non-contiguous regions of the TPS domain to the extracellular β-sheet and loops, and the occurrence of protected species comprising large portions of Fha30 in the proteolysis experiments both support the hypothesis of discrete translocation intermediates. In vitro translocation experiments have also suggested the existence of intermediates [31] . We thus propose that translocation of the TPS domain proceeds by steps of binding, pause and release. The TPS regions that bind strongly to the extracellular sheet in these putative translocation intermediates mainly form extra-β-helix, anti-parallel β-structures in the native TPS domain. Their binding to the FhaC extracellular sheet is thus compatible with the progressive folding of β-helical segments at the surface. The Cys–Cys bonds approach provides a dynamic picture of the FhaC–Fha30 interactions and indicates a funnel-like route for the FHA polypeptide through it transporter. Several crosslinks of a given Fha30 residue with spatially distant residues of FhaC in the POTRA domains and at the barrel entrance indicate >1 possible path(s) as FHA initiates translocation. A major site for POTRA–TPS domain interactions is a hydrophobic groove formed by the edge strand of the β-sheet of the POTRA2 domain and its flanking α-helix, which could accommodate extended, amphipathic segments of the substrate [14] . The highly repetitive, amphipathic structure of the TPS domain [4] , [38] makes it likely that its initial positioning along the POTRA domains is not univocal, and these initial interactions might then determine the entry path of FHA into the channel. As the TPS domain moves through the pore and starts to fold at the surface, it becomes more constrained, and its pathway becomes more defined, as shown by the contacts between the two proteins at the extracellular side of the pore involving exclusively one face of the barrel. We thus propose the following model for the mechanism of secretion. In the absence of its substrate, FhaC transitions from a closed conformation with H1 inside the pore to an open conformation with H1 in the periplasm [23] . The binding of extended amphipathic FHA segments to the POTRA domains of FhaC stabilizes that open conformation and enables the N terminus of FHA to enter and thread its way into the pore. At the exit, specific anti-parallel β-hairpins of the TPS domain of FHA bind to the extracellular β-sheet of FhaC, transiently anchoring the polypeptide at the cell surface and facilitating its folding. Once a sufficient portion of the β-helix is stably formed, backsliding can no longer occur and the rest of the FHA polypeptide progressively emerges and prolongs the β-helix in the extracellular milieu. This scenario is likely to apply to other TPS systems given the good conservation of critical features in both the transporters and the secreted proteins. In the Omp85 superfamily, some members mediate the translocation of their protein substrate across the membrane, whereas others mediate protein insertion into a membrane. However, this distinction is more blurred than generally assumed, and some Omp85 transporters may combine both functions. This is probably the case for TamA and BamA when they secrete autotransporters, which harbour both a transmembrane β-barrel domain and a soluble, extracellular passenger domain [39] , [40] , [41] , [42] . Thus, we believe that some features of the transport process uncovered in this work will be relevant for the other superfamily members. In particular and most importantly, we propose that the direct role for the β-barrel evidenced in this work applies to all Omp85 transporters. This model indeed concurs with mechanisms proposed for BamA and TamA based on recent X-ray structures [11] , [12] , [34] . A lateral opening of the Omp85 β-barrel to enable the transfer of the substrate into the lipid bilayer has been proposed, and evidence supporting such a mechanism was recently obtained [43] . A lateral opening implies that the soluble, surface loop regions of the substrate proteins transit through the barrel while the transmembrane segments are integrated in the bilayer, as discussed in ref. 34 . Those authors have even proposed that the extracellular dome of BamA might function as a lid that restrains misrouting of the substrate membrane strands that might otherwise be secreted [34] . Indeed, the β-strands of these β-barrel substrate proteins are amphipathic, similar to the β-helix-forming segments of TpsA proteins. Unlike the BamA proteins, TamA has no extracellular dome. It has been proposed that the passenger domain of its substrate passes through an enlarged barrel combining those of TamA and the autotransporter, after which the composite barrel splits to release the autotransporter’s barrel into the membrane [12] . The fact that two features of the barrel, L6 and a specific sequence motif in the β-barrel strand B13 are conserved and essential for function [10] , [11] , [25] , [26] corroborates the essential role of the β barrel in the transport process for the entire superfamily. Plasmids pFc3 is the expression plasmid for FhaC [35] . It was modified by site-directed mutagenesis to introduce Cys codons at specific positions using the QuikChange II Xl kit (Agilent Technologies). All mutated fragments were fully verified by sequencing. Deletions were introduced by generating EcoRI–BamHI and BglII–HindIII PCR fragments that encompass the 5′ and 3′ portions of fhaC and ligating them together in EcoRI–HindIII restricted pFc3. Cys codons were introduced into fha30 by site-directed mutagenesis on a modified version of pEC138b (ref. 44 ), harbouring the 3′ NotI–BamHI portion of fha30 made as a synthetic gene fragment (GeneCust) without the PstI site and with codon optimization. To enhance crosslinking, two consecutive Cys codons were introduced together in several Fha30 variants. The relevant restriction fragments were then exchanged for their parent fragments in pEC141bis, which codes for Fha30-BugE (ref. 23 ). The final expression plasmids are based on pBBItac [44] harbouring the EcoRI–HindIII fragments from the corresponding pEC138 and pEC141 variants. pBBItac141b, pBBItac141b-Cmyc and pBBItac-Nmyc for the expression of the Fha30-BugE chimaera and its myc-tagged versions, as well as pBBitac140-calm for the expression of Fha30-calmo were described earlier [23] . In vivo crosslinking E. coli UT5600 cells harbouring both a pFC3 derivative and a pBBItac141b derivative were grown to an OD 600 of 0.8 in 25 ml of LB medium with gentamycin (10 μg ml −1 ) and ampicillin (150 μg ml −1 ) and then treated for 2.5 h with 1 mM IPTG. Cells (4 ml) were harvested by centrifugation, washed once and concentrated 10 times in crosslinking buffer (20 mM HEPES, pH 7.4, 150 mM NaCl and 1 mM EDTA). DMSO or 0.2 mM SPDP, LC-SPDP or SMCC (Thermo Scientific) dissolved in DMSO was added, and the samples were incubated for 1 h at 37 °C under rotation. After quenching for 10 min on ice with 100 mM Tris–HCl (pH 7.5), cells were washed with the crosslinking buffer and lysed by freezing and thawing. The membranes were solubilized in 8 M urea, 1% Triton X-100, 20 mM HEPES (pH 7.4) and 150 mM NaCl. Urea concentration was adjusted to 6 M and the complexes were affinity-purified by incubation with 50 μl of Ni-NTA magnetic beads (Millipore), taking advantage of the natural affinity of FhaC for Ni-NTA. Beads were washed twice in 0.5% Triton X-100, 20 mM HEPES (pH 7.4), 150 mM NaCl containing 6 M urea (washing buffer) and then 2 M urea. The complexes were eluted with 400 mM imidazole in washing buffer. They were resolved by electrophoresis using 3–8% Tris acetate gels (Nu-PAGE—Invitrogen) without reducing agent in the sample buffer and analysed by immunoblotting with polyclonal anti-Fha30 antibodies (dilution 1: 3,000; ref. 23 ) and horseradish peroxidase-coupled anti-guinea pigs antibodies (Jackson ImmunoResearch, catalogue no. 706-035-148; dilution 1:10,000), and the complexes were detected by chemiluminescence. The same blots were then revealed using anti-FhaC antibodies [14] (dilution 1:2,500) and anti-rat alcaline phosphate-conjugated antibodies (Promega, catalogue no. S3831; dilution 1:7,500), followed by colorimetric detection. The contrast of the blot scans for the chemical crosslinking experiments with the chimaera Cys variants was emphasized for better visualization of the complex bands. Cys–Cys crosslinking Cultures were performed as above. Samples of 4 ml were harvested by centrifugation, resuspended in 1 ml PBS containing 5 mM N-ethylmaleimide (Sigma) and incubated for 30 min at room temperature. Cells were then washed in PBS, and membranes were solubilized in 8 M urea, 1% Triton X-100, 20 mM HEPES (pH 7.4), 300 mM NaCl and 1 mM N-ethylmaleimide. Complexes were purified and analysed as described above except that all washing and elution steps were performed in 6 M urea, 0.5% Triton X-100, 20 mM HEPES (pH 7.4) and 300 mM NaCl. The protocol was standardized so that a relative quantification of the complexes could be performed by densitometry scanning of the corresponding bands on the immunoblots using the ImageJ software. Proteolysis Cultures were carried out as above, and 0.7-ml aliquots were centrifuged, washed in PBS and resuspended in 0.6 ml of PBS for intact cells or in 50 mM Tris–HCl (pH 7.5), 10 mM EDTA, 0.1 mg ml −1 lysozyme for outer membrane permeabilization. After 20 min of incubation on ice, proteinase K was added to a final concentration of 500 μg ml −1 , and proteolysis was carried out at 37 °C. Samples of 100 μl were precipitated with TCA after various times, and the proteins were analysed using 12% Tris-glycine gels (Novex, Invitrogen) and immunoblotting with polyclonal anti-Fha30 antibodies [23] or a Myc epitope tag monoclonal antibody (Thermo Scientific, catalogue no. MA1-21316; dilution 1:1,500), followed by secondary horseradish peroxidase-conjugated antibodies as above. For the mass fingerprinting analyses, native Fha30 was purified from culture supernatants [4] and used at a concentration of 20 μg ml −1 . Following proteinase K treatment and electrophoresis, the gel was coloured with Coomassie blue (SimplyBlue Safe Stain, Invitrogen), and the bands of interest were cut and subjected to mass fingerprinting using an Auto Speed TOF/TOF mass spectrometer (Bruker). Flow cytometry analyses Cultures were performed as above, and 1-ml aliquots were harvested at 7,000 r.p.m. for 3 min in a tabletop centrifuge. The cells were washed with ice-cold PBS, 3% BSA, 1% sodium azide and resuspended in 400 μl PBS, 3% BSA, 1% sodium azide containing fluorescein isothiocyanate-conjugated anti-Myc tag antibody (Abcam, catalogue no. 1263; dilution 1:100). After 1 h incubation at room temperature in the dark, cells were pelleted as described above, washed twice in ice-cold PBS with 3% BSA and resuspended in 500 μl of PBS with 3% BSA. Flow cytometry data were acquired on a LSR Fortessa using a photomultiplicator to increase the forward scatter (FSC) signal and analysed with the FACS Diva software (Becton Dickinson). Sequence alignments TpsB proteins were aligned with the Jalview software [45] . How to cite this article: Baud, C. et al . Translocation path of a substrate protein through its Omp85 transporter. Nat. Commun. 5:5271 doi: 10.1038/ncomms6271 (2014).